Coverage enhancement accelerates acidic CO2electrolysis at ampere-level current with high energy and carbon efficiencies Acidic CO 2 electroreduction (CO 2 R) using renewable electricity holds promise for high-efficiency generation of storable liquid chemicals with up to 100% CO 2 utilization. However, the strong parasitic hydrogen evolution reaction (HER) limits its selectivity and energy efficiency (EE), especially at ampere-level current densities. Here we present that enhancing CO 2 R intermediate coverage on catalysts promotes CO 2 R and concurrently suppresses HER. We identified and engineered robust Cu 6 Sn 5 catalysts with strong * OCHO affinity and weak * H binding, achieving 91% Faradaic efficiency (FE) for formic acid (FA) production at 1.2 A cm −2 and pH 1. Notably, the single-pass carbon efficiency reaches a new benchmark of 77.4% at 0.5 A cm −2 over 300 hours. In situ electrochemical Fourier-transform infrared spectroscopy revealed Cu 6 Sn 5 enhances * OCHO coverage ~2.8× compared to Sn at pH 1. Using a cation-free, solid-state-electrolyte-based membrane-electrode-assembly, we produce 0.36 M pure FA at 88% FE over 130 hours with a marked full-cell EE of 37%. The electrochemical reduction of CO 2 (CO 2 R) to valuable short-chain liquid feedstocks presents an elegant solution for storing intermittent renewable electricity, while also mitigating excessive CO 2 emissions resulting from the consumption of fossil fuels [1] , [2] , [3] . In recent decades, significant progress has been made in understanding CO 2 R reaction pathways on catalysts and the associated energetics to control CO 2 R selectivity, and in developing gas-diffusion-electrode-based membrane-electrode-assembly (MEA) electrolyzers capable of achieving industrially relevant CO 2 R current densities over hundreds of mA cm −2 [4] , [5] , [6] , [7] . Despite these efforts, further advancements in CO 2 R technology will depend on improving full-cell energy efficiency (i.e., power-to-product efficiency) and maximizing CO 2 utilization efficiency (i.e., CO 2 -to-product conversion). Operating CO 2 R in acidic electrolytes offers a potential approach to address significant CO 2 losses caused by the reaction between CO 2 and OH − in electrolytes to form CO 3 2− during CO 2 R in alkaline or neutral media. In strong acids with an electrolyte pH ≤ 1, carbonate formation is rare [8] . However, the kinetics of CO 2 R under such highly acidic conditions become retarded. Additionally, the substantial increase in surface * H coverage on catalyst surfaces causes a strong competing hydrogen evolution reaction (HER), resulting in a largely reduced Faradaic efficiency (FE) for CO 2 R [9] , [10] . Early studies have shown that increasing the local concentrations of alkali metal cations in close proximity to catalyst surfaces can enhance CO 2 R by stabilizing the surface-adsorbed CO 2 and CO 2 R-related intermediates through non-covalent interactions, and, at the same time, impeding the diffusion of protons to the catalyst surfaces [11] , [12] , [13] . However, when the system operates at high potentials (i.e. high current densities), the electroconvective flows near the electrodes become turbulent and disordered. According to the Nernst-Planck equation, this turbulence can cause a fluctuation in cation concentrations near the electrode surface, leading to variations in the local electrical field that may have the potential to disrupt the beneficial cation effect on CO 2 R [14] . Prior studies have shown that applying a micrometer-thick layer of nanoparticles as a surface coating layer on catalysts mitigates the irregularities in electroconvective flows within the coated microstructures, which helps maintain a steady concentration profile of alkali metal cations [15] , [16] , [17] . Despite this advancement in mitigating HER, the high local concentration of alkali metal cations can lead to bicarbonate precipitation in the gas diffusion electrodes. The accumulation of bicarbonates hinders CO 2 diffusion and hampers CO 2 R efficiency. To address the bicarbonate precipitation challenge, strategies involve modifying catalysts with immobilized cation groups [18] or exploring CO 2 R in cation-free systems such as using solid-state-electrolyte (SSE) based MEA electrolyzers [19] . One priority for implementing these approaches is to develop efficient catalysts that can inherently promote CO 2 R over the competing HER, particularly under strongly acidic conditions. In this study, we employed computational investigations to discover a Cu 6 Sn 5 catalyst with a notable abundance of surface adsorption sites having a large binding energy difference between * OCHO (the intermediate for formic acid (FA) production) and * COOH (the intermediate for CO production) while also having weaker binding to * H. This configuration allows for maximum selectivity in favor of producing FA over CO and other hydrocarbons while simultaneously suppressing HER. We experimentally constructed Cu 6 Sn 5 alloy catalysts on polytetrafluoroethylene (PTFE) gas diffusion electrodes using thermal vapor deposition. In situ electrochemical attenuated total reflection Fourier-transform infrared (ATR-FTIR) spectroscopy analysis revealed a notable enhancement showcasing a ~2.8 elevation in * OCHO coverage on Cu 6 Sn 5 compared to control catalysts of Sn, operating under identical electrochemical conditions at pH = 1. The active Cu 6 Sn 5 achieves a high FE of 91% for FA production at a current density of 1.2 A cm −2 in a strongly acidic electrolyte at pH = 1. Furthermore, it shows a marked single-pass carbon efficiency (SPCE) of 77.4% at 0.5 A cm −2 , representing approximately 2.8-fold enhancement in the SPCE compared to the prior report of ~27.4% obtained at ~0.24 A cm −2 [20] . Such notable performance was stable over 300 h of continuous acidic CO 2 R at 0.5 A cm −2 in a flow-cell electrolyzer at pH = 1. When integrating Cu 6 Sn 5 into a cation-free, SSE-based MEA electrolyzer, we produced 2.6 liters of 0.36 M pure FA at 100 mA cm −2 (area: 4 cm 2 ) over 130 h at a production rate of 5 mL cm −2 h −1 , along with a full-cell energy efficiency of 37%. These results feature the potential of enhancing surface intermediate coverage as an efficient means for acidic CO 2 R, particularly in cation-free systems at industrially relevant current densities. Density functional theory (DFT) studies Copper (Cu) has established itself as a predominant and cost-effective electrocatalyst capable of generating a variety of hydrocarbons through CO 2 R. Previous research has revealed effective strategies for modifying the * CO-binding and * OCHO-binding properties on surfaces of Cu-based alloy surfaces by introducing foreign elements (e.g., Zn, Al, Pb) into the Cu lattice. Specifically, the inclusion of 5–10 at.% Zn or Al into Cu has shown the ability to partially weaken * CO adsorption on the Al or Zn modified Cu site compared to the adjacent Cu-Cu site, thereby creating asymmetric * CO binding energies for improved C 2+ production [16] , [17] . Additionally, the introduction of a single Pb atom into Cu has been observed to enhance selectivity towards formic acid [21] . These alternations selectively promote the production of CO/C 2+ or FA via distinctive reaction pathways (Fig. 1a ). To further curb the competing HER in strong acids, two major approaches are considered: (1) employing alkali metal cations to hamper H + diffusion toward catalyst surfaces, and (2) augmenting the coverage of surface CO 2 R intermediates to outcompete the HER. Fig. 1: DFT calculations. a Schematic representation of CO 2 R and HER on Cu-based catalysts incorporated with different metal atoms, along with alkali cations effect and coverage enhancement strategy. Color-coded atoms represent Cu (blue), Sn (grey), Zn or Al (yellow), K (purple), O (red), C (brown), and H (pink). b The calculated adsorption energy of * OCHO, * COOH, and * H on Cu, Cu 1− x Sn x ( x = 0.14, 0.44), and Sn catalysts. Since the * H adsorption energies (referring to 1/2 H 2 ) over Cu and Cu 0.86 Sn 0.14 are −0.03 eV and −0.02 eV, it is hard to distinguish their values in the plot. c Differential charge density plots illustrating the enhanced charge transfer between the Cu 6 Sn 5 (−113) surface and * OCHO compared to the other examined surfaces. The isosurface level of the differential charge densities is 0.0045 e/bohr 3 . The yellow or blue areas represent a gain or loss of electrons. Full size image As a representative p-block metal, Sn has a relatively stronger oxygen affinity and weaker adsorption energy for * H than pristine Cu. It can also form alloys with Cu across the entire concentration profile ranging from 0% to 100%. Interestingly, a previous study has investigated the relationship between CO 2 R-to-FA activity and the * OCHO adsorption energy with various metal catalysts [22] , and identified Sn and Cu as promising candidates for selective FA production due to their favorable * OCHO adsorption energies. With this insight, we aimed to create Cu-Sn alloys that could further fine-tune the * OCHO adsorption close to the optimal adsorption-energy values in the adsorption-activity trend. This would contribute to the improvement of the selectivity and activity in the CO 2 R-to-FA conversion. To understand the role of Sn in the Cu 1− x Sn x ( x = 0.14, 0.44) catalysts in tuning the catalytic selectivity of CO 2 R to CO and FA, we built surfaces with various Cu/Sn ratios from pure Cu to Cu 1− x Sn x alloy, and then to pure Sn, and used DFT to calculate the Gibbs free energetic diagrams for CO and FA generation. Based on the previous literature reviews [23] , [24] , the potential rate-determining step (RDS) for the CO 2 R-to-CO conversion is the first proton transfer to form * COOH from CO 2 (CO 2 (gas) + H + + e − + * → * COOH), while the potential RDS for CO 2 R-to-FA is the first proton transfer to form * OCHO (CO 2 (gas) + H + + e − + * → * OCHO). By using DFT calculations, we identified that the Cu 6 Sn 5 alloy possesses a high abundance of surface sites with a stronger binding affinity to * OCHO compared to * COOH, making it thermodynamically more favorable for producing FA (Fig. 1b ). In addition, Cu 6 Sn 5 exhibits notably weaker binding to * H ( + 0.33 eV referring to 1/2 H 2 ), resulting in a substantial energy requirement for H 2 production and thus, suppressing HER. To study how the electronic properties of the surface-active sites on Cu 1− x Sn x catalysts with varying Sn concentrations affect the selectivity of FA and CO production, we calculated the differential charge density of * OCHO and * COOH over the experimentally observed surfaces in Fig. 1c . Our results indicate that the Cu 6 Sn 5 (−113) surface exhibits more charge transfer with * OCHO than that over other examined surfaces. This charge analysis is consistent with the adsorption energy calculation, where the Cu 6 Sn 5 (−113) surface exhibits the strongest adsorption energy of * OCHO among all the examined surfaces. Such strong adsorption energy of * OCHO also indicates a potentially high surface coverage of * OCHO over the Cu 6 Sn 5 (−113) surface. In addition, since two O−Cu bonds are formed between O δ− of * OCHO and Cu atoms on Cu 1− x Sn x surfaces, our results show that Cu 6 Sn 5 (−113) surface presents ~1.3 and ~2.3 eV more favorable formation energy for * OCHO than for * COOH under alkaline (Supplementary Fig. 1 ) and acidic (Fig. 2a ) conditions, respectively. Furthermore, according to the experimental results in Fig. 2b , the production of C 2+ and CH 4 products disappeared over the metal surface when the concentration of Sn in Cu 1− x Sn x catalysts was increased to ~14%. To reveal the role of Sn in Cu 1− x Sn x catalysts in eliminating the C 2+ and CH 4 production during CO 2 R, we compared the adsorption energy of CO over pure Cu (111) and Cu 0.86 Sn 0.14 (111) surfaces (Supplementary Fig. 2 ). The DFT results show that the presence of Sn on the Cu 0.86 Sn 0.14 (111) surface weakens the adsorption of CO to ~0 eV compared to −0.08 eV on the pure Cu (111) surface. Thus, CO will likely desorb from the Cu 0.86 Sn 0.14 (111) surface and be unable to hydrogenate via H protonation to produce CH 4 or couple with another adsorbed * CO intermediate to generate C 2+ species. These findings are in agreement with previous literature reports and experiments that have observed no C 2+ and CH 4 species produced over Cu 0.86 Sn 0.14 [25] , [26] . Fig. 2: Electrochemical performance of CO 2 reduction with Cu, Cu 1− x Sn x ( x = 0.08, 0.14, 0.28, 0.44, 0.71, 0.88) and Sn catalysts in 3 M KCl and 0.05 M H 2 SO 4 electrolyte at pH 1 in flow cells. a A volcano-like plot showing the Gibbs free energy difference (ΔG) between * OCHO (an intermediate for FA production) and * COOH (an intermediate for CO production) over Cu (111), Cu 0.86 Sn 0.14 (111), Cu 6 Sn 5 (−113), and Sn (100) surfaces. This plot is in line with the obtained experimental data of Faradaic efficiency (FE) for FA production at 1.2 A cm −2 in 3 M KCl and 0.05 M H 2 SO 4 . Gibbs free energy was calculated at room temperature (298.15 K), pH of 1, and an applied potential of −2.1 V vs. reversible hydrogen electrode (V RHE ) using computational hydrogen electrode (CHE) model. b Distributions of Faradaic efficiencies (FE) for formic acid (FA), H 2 , C 2+ , CO, and CH 4 at 0.1, 0.4, 0.8, 1.2, and 1.6 A cm −2 . The error bars presented are derived from three independent tests. c Partial current densities of FA as a function of the applied potentials on Cu, Cu 1− x Sn x ( x = 0.08, 0.14, 0.28, 0.44, 0.71, 0.88), and Sn catalysts. d Single-pass carbon efficiency (SPCE) of CO 2 R on Cu 6 Sn 5 at 0.5 A cm −2 , obtained at pH 1 and 14 at different CO 2 flow rates of 3, 6, 10, 15, 18.5 standard cubic centimeter per minute (sccm). The error bars presented are derived from three independent tests. e Performance comparison of this study and the previously published data under acidic conditions. Full size image We performed Gibbs free energy calculations to quantitatively determine the reaction energy difference between the reaction pathways of CO 2 – * COOH–CO/C 2+ and CO 2 – * OCHO–HCOO − over the experimentally observed surfaces, including Cu (111), Cu 0.86 Sn 0.14 (111), Cu 6 Sn 5 (−113), and Sn (100) surfaces, where the possible reaction mechanisms have been shown in Supplementary Fig. 3 . These calculated surfaces are the dominant facets in XRD measurement in Supplementary Figs. 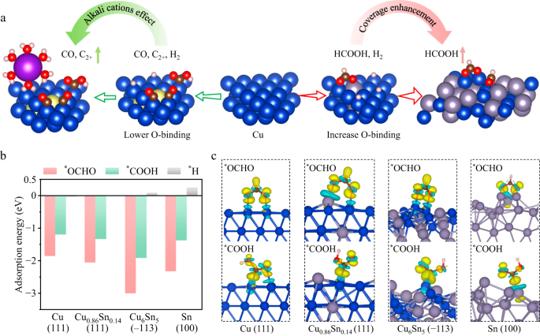Fig. 1: DFT calculations. aSchematic representation of CO2R and HER on Cu-based catalysts incorporated with different metal atoms, along with alkali cations effect and coverage enhancement strategy. Color-coded atoms represent Cu (blue), Sn (grey), Zn or Al (yellow), K (purple), O (red), C (brown), and H (pink).bThe calculated adsorption energy of*OCHO,*COOH, and*H on Cu, Cu1−xSnx(x= 0.14, 0.44), and Sn catalysts. Since the*H adsorption energies (referring to 1/2 H2) over Cu and Cu0.86Sn0.14are −0.03 eV and −0.02 eV, it is hard to distinguish their values in the plot.cDifferential charge density plots illustrating the enhanced charge transfer between the Cu6Sn5(−113) surface and*OCHO compared to the other examined surfaces. The isosurface level of the differential charge densities is 0.0045 e/bohr3. The yellow or blue areas represent a gain or loss of electrons. 4 – 9 and Supplementary Table 1 . Gibbs free energetic diagrams for the formation of * OCHO and * COOH over different catalytic surfaces were constructed according to the experimental conditions of room temperature, pH 1 of the electrolyte, and an applied potential of −2.1 V vs. RHE (V RHE ). Our theoretical results (Fig. 2a , Supplementary Figs. 10 – 33 ) show that the Gibbs free energy differences (ΔG = G( * COOH) − G( * OCHO)) of the potential RDSs of FA and CO pathways during CO 2 R present a volcano-like plot as increasing the concentration of Sn in the Cu 1− x Sn x catalysts. Among the four examined surfaces, Cu 6 Sn 5 (−113) shows the largest ΔG between the CO 2 R to FA and CO pathways, indicating that Cu 6 Sn 5 (−113) contributes the highest selectivity for FA production. The theoretical results are consistent with the experimental results (Fig. 2b , c ) that the FE of FA production over Cu 6 Sn 5 is the highest. To examine the competitive HER over Cu (111), Cu 0.86 Sn 0.14 (111), Cu 6 Sn 5 (−113) and Sn (100) surfaces, we examined the energy diagram of HER (Supplementary Fig. 34 ). The corresponding * H adsorption configurations can be seen in Supplementary Figs. 35 – 38 . The increased free energy of HER indicates that the HER will be suppressed, and the selectivity for CO 2 R can thus be improved over Cu 0.86 Sn 0.14 , Cu 6 Sn 5 , and Sn compared to that on pristine Cu. This is consistent with experimental results (Fig. 2b ), which show the FE of HER over Cu is higher than that on Cu 0.86 Sn 0.14 , Cu 6 Sn 5 , and Sn. Finally, we built surfaces with different Cu/Sn ratios, ranging from pure Cu to Cu 1− x Sn x alloy, and then to pure Sn. Using DFT calculations, we analyzed the surface formation energetics for each surface. As depicted in Supplementary Fig. 39 , Cu 6 Sn 5 (−113) shows improved stability with a lower surface formation energy compared to the pristine Cu (111) facet. Conversely, Sn (100) shows poor stability with a higher surface formation energy. Electrochemical CO 2 R studies With the theoretical insight, we conducted a systematical investigation into the Cu–Sn alloy as an illustrative catalyst system with the objective of obtaining exclusive CO 2 R to HCOOH at high current densities while also achieving high energy and carbon efficiencies. Experimentally, we created Cu 1− x Sn x ( x = 0.08, 0.14, 0.28, 0.44, 0.71, 0.88) and control catalysts of pure Cu and Sn on PTFE gas diffusion electrodes using thermal evaporation (Supplementary Figs. 4 and 40 , 41 ). We evaluated their CO 2 R performance for Cu 1− x Sn x ( x = 0.08, 0.14, 0.28, 0.44, 0.71, 0.88) and controlled Cu and Sn catalysts in a flow cell with a three-electrode configuration in both alkaline and acid electrolytes. We quantitatively analyzed the gas and liquid products using gas chromatography (GC), nuclear magnetic resonance spectroscopy (NMR), and ion chromatography (IC). In a 1 M KOH electrolyte at pH 14, the linear sweep voltammetry (LSV) curves in Supplementary Fig. 42 showed a sharp increase in the current densities with the increase of applied negative potentials, indicating efficient electrical conductivity for the Cu and Cu 1− x Sn x ( x < 0.71) electrodes. With the addition of Cu in Cu 1− x Sn x ( x < 0.71), the onset potential for formate shifted positively, indicating improved CO 2 R kinetics. At high current densities, Cu 6 Sn 5 also displayed the highest selectivity for formate production, with over 90% formate FEs across a wide current density range of 0.4 to 1.2 A cm −2 (Supplementary Fig. 43 ). The Cu 6 Sn 5 catalyst showed formate partial current densities of up to ~1.5 A cm −2 at a relatively low operating potential of around −1.8 V RHE (Supplementary Fig. 44 ) and the highest formate selectivity close to 90% (Supplementary Fig. 43 ). To assess the stability of Cu 6 Sn 5 in 1 M KOH, we carried out Galvanostatic tests using an alternating current density mode (0.05 A cm −2 for 30 s and 0.5 A cm −2 for 90 s) [17] for 160 hours in a flow cell (Supplementary Fig. 45 ). Prior to the stability test, we coated a carbon-Nafion™ or SiC-Nafion™ mixed layer with a thickness of 2–5 μm on the surface of Cu 6 Sn 5 to enable a uniform electrohydrodynamic flow near the catalysts [14] . Through the 120-h CO 2 R operation at a current density of 0.5 A cm −2 , we obtained a stable formate FE of above 85%. When comparing the FE and current density of this work with the previous reports under alkaline conditions, we found that we found that our results are superior (Supplementary Fig. 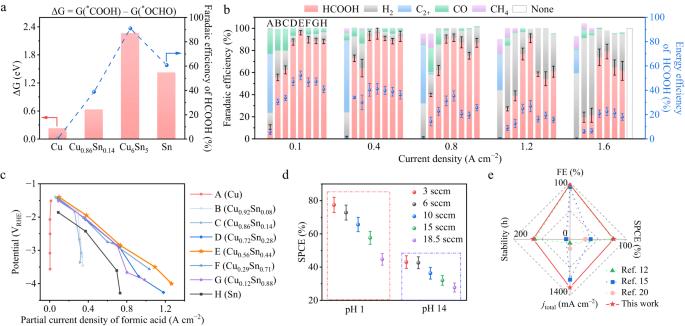Fig. 2: Electrochemical performance of CO2reduction with Cu, Cu1−xSnx(x= 0.08, 0.14, 0.28, 0.44, 0.71, 0.88) and Sn catalysts in 3 M KCl and 0.05 M H2SO4electrolyte at pH 1 in flow cells. aA volcano-like plot showing the Gibbs free energy difference (ΔG) between*OCHO (an intermediate for FA production) and*COOH (an intermediate for CO production) over Cu (111), Cu0.86Sn0.14(111), Cu6Sn5(−113), and Sn (100) surfaces. This plot is in line with the obtained experimental data of Faradaic efficiency (FE) for FA production at 1.2 A cm−2in 3 M KCl and 0.05 M H2SO4. Gibbs free energy was calculated at room temperature (298.15 K), pH of 1, and an applied potential of −2.1 V vs. reversible hydrogen electrode (VRHE) using computational hydrogen electrode (CHE) model.bDistributions of Faradaic efficiencies (FE) for formic acid (FA), H2, C2+, CO, and CH4at 0.1, 0.4, 0.8, 1.2, and 1.6 A cm−2. The error bars presented are derived from three independent tests.cPartial current densities of FA as a function of the applied potentials on Cu, Cu1−xSnx(x= 0.08, 0.14, 0.28, 0.44, 0.71, 0.88), and Sn catalysts.dSingle-pass carbon efficiency (SPCE) of CO2R on Cu6Sn5at 0.5 A cm−2, obtained at pH 1 and 14 at different CO2flow rates of 3, 6, 10, 15, 18.5 standard cubic centimeter per minute (sccm). The error bars presented are derived from three independent tests.ePerformance comparison of this study and the previously published data under acidic conditions. 46 and Supplementary Table 2 ) [6] , [11] , [19] , [21] , [27] , [28] , [29] , [30] , [31] , [32] , [33] , [34] , [35] , [36] , [37] , [38] , [39] , [40] , [41] , [42] , [43] , [44] . In 3 M KCl and 0.05 M H 2 SO 4 electrolyte at pH 1, Cu 6 Sn 5 exhibited the highest selectivity, reaching up to 96% at −1.4 V RHE for formic acid in Fig. 2c . Remarkably, Cu 6 Sn 5 showed a high FE of above 90% for FA production across a wide range of current densities from 0.4 to 1.2 A cm −2 (Fig. 2b ). We examined the SPCE for Cu 6 Sn 5 under a constant current density of 0.5 A cm −2 in a flow cell equipped with a 1.7 × 1.7 cm 2 serpentine channel reaction area at various CO 2 flow rates and electrolyte pH levels (more details are presented in the Supplementary Information) [15] . Figure 2d presents a maximum SPCE of 77.4%, achieved at a CO 2 flow rate of 3 standard cubic centimeter per minute (sccm) under pH 1 conditions. The electrode of Cu 6 Sn 5 coated with carbon-Nafion™ or SiC-Nafion™ demonstrated stable FA production for over 300 hours, maintaining over 70% FE at a cathodic potential of −2.5 V RHE . This equated to a 40% cathodic energy efficiency (CEE) at 0.5 A cm −2 at pH 1 (Supplementary Fig. 47 ). Theoretical investigations were correspondingly carried out in this segment to investigate the effects of the electrochemical operating environment effects (e.g., electrolyte of 3 M K + , applied potential of −2.1 V RHE , and pH = 1) on the selectivity for FA vs. CO formation using Constant Electrode Potential (CEP) model via performing Grand canonical DFT calculations [45] , [46] , [47] , [48] , [49] . The selectivity for FA across Cu (111), Cu 0.86 Sn 0.14 (111), Cu 6 Sn 5 (−113), and Sn (100) surfaces exhibits a volcano plot (Fig. 2a and Supplementary Fig. 48 ), with Cu 6 Sn 5 (−113) displaying the highest energy difference between the two pivotal intermediates, favoring the adsorption of * OCHO over CO. More details regarding grand canonical DFT simulations are provided in Supplementary Information. We compared this work with previously reported results on the CO 2 R-to-FA production under acidic conditions in terms of elevated current density, FE, SPCE, and stability in Fig. 2e [12] , [15] , [20] . Characterization We conducted material and structure characterizations, as well as surface wettability analysis, for the Cu 6 Sn 5 catalyst before the CO 2 R reaction. 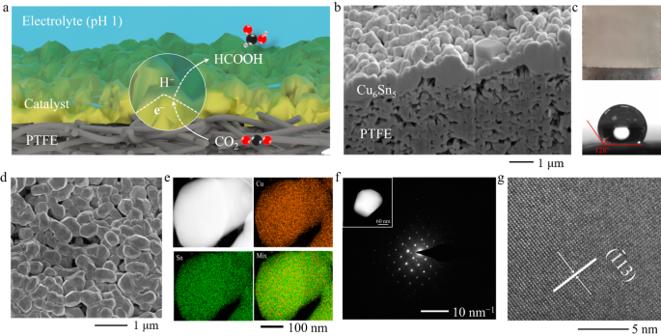Fig. 3: Characterizations of the thermally evaporated Cu6Sn5-on-PTFE electrodes. aSchematic representation of the CO2R process on Cu6Sn5-on-PTFE electrodes.bCross-sectional SEM image of the Cu6Sn5/PTFE electrode, showcasing the dense arrangement of Cu6Sn5nano-to-micro particles on the PTFE substrate.cOptical image and the measured contact angle of a water droplet on the Cu6Sn5-on-PTFE electrode.d–gTop-view SEM image (d), STEM-EDX images (e), HAADF image and SAED pattern (f), and HRTEM image (g) of the thermally evaporated Cu6Sn5catalyst. Figure 3a shows a schematic of the CO 2 R process on Cu 6 Sn 5 /PTFE electrodes. The cross-sectional scanning electron microscope (SEM) image in Fig. 3b shows the well-defined structure of Cu 6 Sn 5 nano-to-micro particles densely packed on the PTFE substrate. This Cu 6 Sn 5 -on-PTFE structure was synthesized over a large scale via thermal evaporation (Fig. 3c and Supplementary Fig. 49 ), exhibiting hydrophobicity, as indicated by a water contact angle of 128° (Fig. 3c ). This hydrophobicity enables CO 2 diffusion through the gaps between the particles on the PTFE sides to the catalyst surface (Fig. 3a ). The top-view SEM presents that the diameter of the Cu 6 Sn 5 particles is 300–600 nm (Fig. 3d ). Energy dispersive X-ray spectroscopy in transmission electron microscopy (STEM-EDX) analysis revealed a uniform distribution of Sn and Cu over the majority of the Cu 6 Sn 5 particles (Fig. 3e ). Fig. 3: Characterizations of the thermally evaporated Cu 6 Sn 5 -on-PTFE electrodes. a Schematic representation of the CO 2 R process on Cu 6 Sn 5 -on-PTFE electrodes. b Cross-sectional SEM image of the Cu 6 Sn 5 /PTFE electrode, showcasing the dense arrangement of Cu 6 Sn 5 nano-to-micro particles on the PTFE substrate. 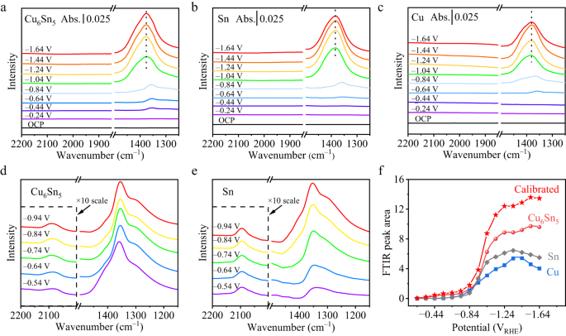Fig. 4: In situ ATR-FTIR spectroscopy analysis. a–cIn situ ATR-FTIR spectra measured at different applied potentials for Cu6Sn5(a), Sn (b), and Cu (c) under identical electrochemical conditions at pH = 1. Abs. stands for absorbance.d,eATR-FTIR results of Cu6Sn5(d), and Sn (e) in the potential range of −0.54 to −0.94 VRHE, which were used to calculate the relative peak areas of*OCHO using the peak areas of the potassium ferricyanide as a reference. The peak intensities of the internal standard potassium ferricyanide in panels (d) and (e) have been magnified by 10 times to facilitate comparison with those of the*OCHO intermediates.fThe integrated ATR-FTIR peak areas of the Cu, Sn, Cu6Sn5with and without calibration. c Optical image and the measured contact angle of a water droplet on the Cu 6 Sn 5 -on-PTFE electrode. d – g Top-view SEM image ( d ), STEM-EDX images ( e ), HAADF image and SAED pattern ( f ), and HRTEM image ( g ) of the thermally evaporated Cu 6 Sn 5 catalyst. Full size image Detailed structural analysis using transmission electron microscope (TEM), high-resolution transmission electron microscope (HRTEM), and selective area electron diffraction (SAED) analyses (Fig. 3f , g ) confirmed the formation of monoclinic Cu 6 Sn 5 crystal. These results are in line with the X-ray powder diffraction (XRD) patterns in Supplementary Fig. 50 , which indicate the presence of the main (−113), (132), and (−314) facets for Cu 6 Sn 5 . More details regarding the crystallographic and material analysis of catalysts after acidic CO 2 R operation are presented in Supplementary Figs. 51 – 53 . In situ ATR-FTIR analysis We used in situ ATR-FTIR spectroscopy to study CO 2 R intermediates coverage on Cu 6 Sn 5 -on-PTFE, Cu-on-PTFE, and Sn-on-PTFE electrodes during acidic CO 2 R electrolysis in the same pH 1 electrolyte of 3 M KCl and 0.05 M H 2 SO 4 , spanning a range of applied potentials from −0.24 to −1.64 V RHE . We also incorporated an internal standard of potassium ferricyanide in the electrolytes to facilitate peak area calibration. In the ATR-FTIR spectra for the Cu 6 Sn 5 and Sn catalysts (Fig. 4a – c ), significant peaks were absent within the range of 1900 to 2200 cm −1 . In contrast, distinct infrared vibration bands related to the * OCHO intermediate were observed within the 1375–1385 cm −1 range for all Cu 6 Sn 5 , Cu, and Sn catalysts. The onset potential for the * OCHO intermediate on Cu 6 Sn 5 was −0.44 V RHE , lower than that on Cu and Sn, indicating fast CO 2 R-to-HCOOH kinetics with Cu 6 Sn 5 . During the in situ ATR-FTIR test using a 5 mM potassium ferricyanide internal standard in 3 M KCl and 0.05 M H 2 SO 4 , we observed a constant peak area for potassium ferricyanide within the potential range of −0.54 to −0.94 V RHE . Consequently, we established a calibration curve within this potential range, using the potassium ferricyanide peak as a reference. This allowed us to calculate the peak areas of * OCHO intermediates on different catalysts at the same potential range (Fig. 4d , e and Supplementary Table 3 ). Notably, adhering the established calibration relationship, the plateau * OCHO peak intensity on Cu 6 Sn 5 measured at potentials above −1.04 V RHE in the CO 2 R electrolyte is ~2.8 times higher than that of Sn, with all measurements conducted under identical conditions (Fig. 4f ). These results point toward an enhanced surface coverage of * OCHO on Cu 6 Sn 5 , which facilitates selective FA production during acidic CO 2 R. Fig. 4: In situ ATR-FTIR spectroscopy analysis. a – c In situ ATR-FTIR spectra measured at different applied potentials for Cu 6 Sn 5 ( a ), Sn ( b ), and Cu ( c ) under identical electrochemical conditions at pH = 1. Abs. stands for absorbance. d , e ATR-FTIR results of Cu 6 Sn 5 ( d ), and Sn ( e ) in the potential range of −0.54 to −0.94 V RHE , which were used to calculate the relative peak areas of * OCHO using the peak areas of the potassium ferricyanide as a reference. The peak intensities of the internal standard potassium ferricyanide in panels ( d ) and ( e ) have been magnified by 10 times to facilitate comparison with those of the * OCHO intermediates. f The integrated ATR-FTIR peak areas of the Cu, Sn, Cu 6 Sn 5 with and without calibration. Full size image To produce a pure formic acid solution, we conducted CO 2 R using an AEM (Sustainion X37-50 Grade) based SSE-MEA electrolyzer. 0.5 M H 2 SO 4 was used as the anolyte and IrO x /Ti foam was used as the anode (Fig. 5a ). During the electrolysis, HCOO − was generated on the cathode side and diffused through the AEM into the middle SSE layer. Simultaneously, H + permeated through the CEM (Nafion 117) and reacted with HCOO − to form FA. The produced FA solution was collected by passing deionized water through the SSE layer. As shown in Fig. 5a , the operating potential is 3.4 V for the overall CO 2 -to-FA and H 2 O-to-O 2 reaction in an SSE-based MEA electrolyzer. The detailed potential distributions are listed in Fig. 5a : a theoretical potential of 1.43 V required to initiate the CO 2 R-to-FA reaction, a ~0.3 V overpotential on the IrO x loaded Ti mesh anode, and an ~1.5 V overpotential on the SSE, anion and cation membranes, and Cu 6 Sn 5 cathode. In Fig. 5b , using the Cu 6 Sn 5 catalyst, the FA FE reached ~96% at 100 mA cm −2 . The full-cell voltage was −3.7 V and the full-cell energy efficiency was over 37%. We evaluated the CO 2 R performance in different anolytes (0.1 M, 0.5 M, and 1 M H 2 SO 4 ) in Supplementary Fig. 54 . We quantified the amount of FA produced using IC, NMR, and pH measurements (Supplementary Fig. 55 ). The results confirmed the production of 2.6 liters of 0.36 M pure FA solution (Supplementary Fig. 56 ) with a production rate of 5 mL cm −2 h −1 (20 mL h −1 ) over a continuous 130-h CO 2 R process (Fig. 5c ). 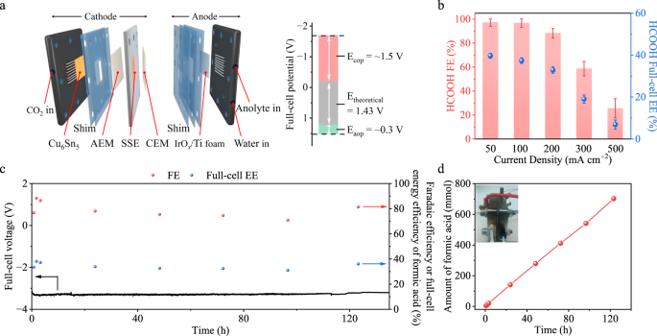Fig. 5: Electrochemical CO2R performance with Cu6Sn5in acidic electrolytes at pH 1. aStructure of a solid-state-electrolyte-based membrane electrode assembly electrolyzer for CO2R and its potential distribution.bFEs and full-cell energy efficiencies of FA production with Cu6Sn5at different current densities. The error bars presented are derived from three independent tests.cFEs and full-cell energy efficiencies of FA production with Cu6Sn5at 100 mA cm−2during 130-h CO2R operation.dOptical image of MEA and production rate of FA with Cu6Sn5at 100 mA cm−2during 130-h CO2R operation. Figure 5d shows an optical image of an SSE-based MEA and a steady production rate of FA over the 130-h CO 2 R process to produce ~700 mmol pure FA. Fig. 5: Electrochemical CO 2 R performance with Cu 6 Sn 5 in acidic electrolytes at pH 1. a Structure of a solid-state-electrolyte-based membrane electrode assembly electrolyzer for CO 2 R and its potential distribution. b FEs and full-cell energy efficiencies of FA production with Cu 6 Sn 5 at different current densities. The error bars presented are derived from three independent tests. c FEs and full-cell energy efficiencies of FA production with Cu 6 Sn 5 at 100 mA cm −2 during 130-h CO 2 R operation. d Optical image of MEA and production rate of FA with Cu 6 Sn 5 at 100 mA cm −2 during 130-h CO 2 R operation. Full size image In this study, we demonstrate the effectiveness of enhancing surface coverage of CO 2 R intermediates as a strategy to promote CO 2 R at ampere-level current densities and under strongly acidic conditions. Theoretical DFT calculations have revealed that Cu 6 Sn 5 enhances the adsorption of * OCHO compared to * COOH and * H, resulting in increased surface * OCHO coverage and promoted FA production in CO 2 R while simultaneously suppressing the HER. Experiments have identified a robust Cu 6 Sn 5 catalyst that exhibits exclusive FA production with over 90% FE at 1.2 A cm −2 , and a remarkable 77.4% carbon efficiency at 0.5 A cm −2 , maintaining stability over 300 h of continuous CO 2 R operation at pH = 1. In situ electrochemical ATR-FTIR spectroscopy validates an approximately 2.8× enhancement in * OCHO coverage on Cu 6 Sn 5 compared to the control catalyst of Sn, operating under identical electrochemical conditions at pH = 1. Furthermore, using an SSE-based MEA electrolyzer, we stably produce pure FA solution with a concentration of 0.36 M over a 130-hour reaction at a full-cell energy efficiency surpassing 37%. We expect that the insights gained from our work, particularly in the context of optimizing intermediate adsorption and coverage, will provide valuable guidance for the advancement of selective and energy-efficient CO 2 R with long-lasting performance in cation-free, MEA-based electrolyzers. Density functional theory (DFT) calculation DFT calculations were conducted using the Vienna Ab-initio Simulation Package (VASP) [50] . To take the solvation effects into consideration, hybrid solvation effects have been employed in VASPsol along with explicit water molecules at the interface [45] , [46] , [47] , [48] . The Constant Electrode Potential (CEP) model has been employed to investigate the constant negative applied potential and cation effects through grand-canonical DFT (GC-DFT) calculations [49] . These calculations were used to compare the energy diagrams of two possible CO 2 reduction reaction (CO 2 R) pathways over different surfaces. We have investigated Cu (111), Cu 0.86 Sn 0.14 (111), Cu 6 Sn 5 (−113), and Sn (100) surfaces for calculations (Supplementary Fig. 4 ), where these facets are also the most thermodynamic favorable ones for Cu, Sn, and Cu 1− x Sn x alloy systems. More DFT calculation details are included in the Supplementary Information. Synthesis We fabricated a series of Cu 1− x Sn x ( x = 0.08, 0.14, 0.28, 0.44, 0.71, 0.88), Cu, and Sn electrocatalysts by thermal evaporation (SKY-RH400). Cu and Sn particles were placed separately in two Molybdenum boats inside the deposition chamber and melted slowly under the pressure of 10 −5 Torr for thermal evaporation. We controlled the thermal evaporation rates of Cu and Sn to adjust the Cu/Sn ratios in the synthesized alloys. Evaporating rates of approximately x Å s −1 ( x = 0.08, 0.14, 0.28, 0.44, 0.71, 0.88) for Sn and approximately (1− x ) Å s −1 for Cu were used to produce alloyed Cu 1− x Sn x films on the polytetrafluoroethylene (PTFE) substrates. A quartz crystal monitor was used to observe the thicknesses of evaporated Cu 1− x Sn x . Evaporation of pure Sn and pure Cu electrocatalysts was conducted using a similar fabrication procedure. The loading of all catalysts is 800 nm thick. Characterization Transmission electron microscopy (SEM) images were taken using a Hitachi SU8100 SEM at an accelerating voltage of 5 kV. High-resolution transmission electron microscopy (HRTEM) and transmission electron microscopy-energy dispersive X-ray spectroscopy (TEM-EDX), selected area electron diffraction (SAED), and bright-field and dark-field TEM analyses were performed in a TEM (Tecn F20) with an accelerating voltage of 200 kV. X-ray powder diffraction (XRD) was carried out with a Bruker D8 Advance at a scanning rate of 10° min −1 in the 2θ range from 20° to 80°. X-ray photoelectron spectroscopy (XPS) studies were performed using PHI5000 VersaProbe. The binding energy data were calibrated relative to the C 1 s signal at 284.6 eV. Electrochemical experiments Experiments under alkaline and acidic conditions were performed in a flow cell using a three-electrode system. Ag/AgCl electrode was used as the reference electrode, commercial Ni foam (for use under alkaline conditions) and Pt (for use under acidic conditions) were used as the counter electrodes, Cu 1− x Sn x ( x = 0.08, 0.14, 0.28, 0.44, 0.71, 0.88), Cu, and Sn on PTFE electrodes were used as the working electrodes (area: 0.5 cm 2 ), and the electrolytes were 1 M KOH (for alkaline CO 2 electrolysis) and 0.05 M H 2 SO 4 with 3 M KCl (for acidic CO 2 electrolysis). Anion exchange membrane (Fumasep FAB-PK-130, size: 2 × 2 cm 2 , thickness: 130 μm) and proton exchange membrane (Nafion N117, size: 2 × 2 cm 2 , thickness: 183 μm) were used as the ion exchange membranes. The proton exchange membrane was immersed in 0.5 M H 2 SO 4 for about 2 h before use. Experiments using solid-state electrolyte (SSE) were performed in a membrane electrode assembly (MEA) system with a 1 mm-thick SSE layer between the cathode and anode. IrO x /Ti foam was used as the anode, and Cu 6 Sn 5 was used as the cathode (area: 4 cm 2 ). Anion exchange membrane (Sustainion X37-50 Grade, size: 4 × 4 cm 2 , thickness: 50 μm) and proton exchange membrane (Nafion N117, size: 4 × 4 cm 2 , thickness: 183 μm) were used as the ion exchange membranes. The SSE was AmberChrom 50WX4 hydrogen form (J&K Scientific), and the anolyte was 0.5 M H 2 SO 4 . The electrochemical workstation was Autolab PGSTAT302N (Metrohm). The gas flow rate was controlled at 25 mL min −1 by an electronic flow meter, and the end flow rate was calibrated by a soap film flow meter during the test. All of the electrode potentials vs. the Ag/AgCl electrode were converted to the potentials vs. reversible hydrogen electrode (RHE) using the following Eq. ( 1 ): 
    E_RHE=E_Ag/AgCl+0.197+0.059×pH+iR
 (1) Gas-phase products were measured using gas chromatography (GC Agilent 990, Perkin Elmer Clarus 680). According to the peak area, the Faradaic efficiency of the gas products can be obtained, and the calculation formula is as the following Eq. ( 2 ): 
    FE=F× z× v× n/I× t× 100%
 (2) where F is the Faraday’s constant, which is 96485 C mol −1 . z is the number of electrons required to reduce CO 2 to a CO or H 2 molecule, which is 2. v is the gas flow rate, here is 25 mL min −1 . n is the concentration of the gas products obtained by GC with 1 mL of sample gas, the unit is mol mL −1 . I is the current applied to the sample, the unit is A. t is the reaction time, and the unit is s. Liquid product HCOO − was measured using ion chromatography (IC, SH-AC-11, Qingdao shenghan). The FE towards formate or FA at each current density was calculated by adding up both anodic and cathodic FEs. We first obtained a standard curve with a concentration gradient of sodium formate (HCOONa), HCOO − concentrations were set as 1 ppm, 2 ppm, 5 ppm, 10 ppm, 50 ppm, and 100 ppm (mg L −1 ). According to this, the HCOO − concentration in the electrolyte after the reaction can be obtained. The formula of faradaic efficiency calculation for HCOO − is as the following Eq. ( 3 ): 
    FE=F× z× V× n/45× I× t× 100%
 (3) where F is the Faraday’s constant, which is 96485 C mol −1 . n is the concentration of HCOO − measured by the instrument based on the standard curve, and the unit is mg L −1 . z is the number of electrons required for the reduction of CO 2 into HCOO − , here is 2. V is the volume of the catholyte, here is 0.03 L. t is the reaction time, and the unit is s. All data, including Faradaic efficiencies, were collected based on 1-hour electrolysis. Stability tests were conducted over 300 h. The overpotential is determined by subtracting the operating potential at specific current densities for formic acid generation from the theoretic potential for formic acid production, which is −0.199 V RHE . In situ electrochemical attenuated total reflection Fourier-transform infrared spectroscopy (ATR-FTIR) experiments were conducted on a Thermo Scientific Nicolet 6700 FTIR spectrometer with ZnSe as the prismatic window at room temperature. A three-electrode electrochemical single-cell was used for the tests (Supplementary Fig. 57 ). The thermally-evaporated Cu 6 Sn 5 catalyst on a carbon gas diffusion layer (Freudenberg H15C13) was used as the working electrode, a Pt wire was used as the counter electrode, and a saturated Ag/AgCl electrode was used as the reference electrode. 3 M KCl and 0.05 M H 2 SO 4 (pH = 1) saturated with CO 2 was used as the electrolyte. Open circuit potential (OCP) was conducted as a comparison, and the data was collected using chronoamperometric tests from −0.24 to −1.64 V RHE . The peak area of * OCHO in FTIR was calculated by integrating the corresponding curve areas in the same interval (1250–1500 cm −1 ) obtained at different potentials. More experimental details are discussed in the Supplementary Information.